Bloch oscillations in plasmonic waveguide arrays The combination of modern nanofabrication techniques and advanced computational tools has opened unprecedented opportunities to mold the flow of light. In particular, discrete photonic structures can be designed such that the resulting light dynamics mimics quantum mechanical condensed matter phenomena. By mapping the time-dependent probability distribution of an electronic wave packet to the spatial light intensity distribution in the corresponding photonic structure, the quantum mechanical evolution can be visualized directly in a coherent, yet classical wave environment. On the basis of this approach, several groups have recently observed discrete diffraction, Bloch oscillations and Zener tunnelling in different dielectric structures. Here we report the experimental observation of discrete diffraction and Bloch oscillations of surface plasmon polaritons in evanescently coupled plasmonic waveguide arrays. The effective external potential is tailored by introducing an appropriate transverse index gradient during nanofabrication of the arrays. Our experimental results are in excellent agreement with numerical calculations. The dynamics of waves in structured potentials plays an important role in many branches of physics—for example, solid-state physics, atomic physics, photonics or acoustics. Despite the different natures of these waves, the corresponding equations that govern their evolution can have the same mathematical form and hence allow mapping of wave phenomena in different physical systems on each other. This is the key idea behind the emerging field of quantum simulators [1] , [2] , where the quantum dynamics of a system that is hardly accessible by experimental means is reproduced with other equivalent quantum or classical optical systems [3] , [4] , providing a much better experimental control over the relevant parameters. For example, Felix Bloch predicted in his seminal paper [5] that a crystal electron carries out an oscillatory motion under the influence of an external static electric field. While scattering of the electron prevents Bloch oscillations in bulk crystals, they have been observed in a number of equivalent systems, such as semiconductor superlattices [6] , atomic systems [7] , [8] , arrays of coupled dielectric waveguides [9] , [10] and periodic dielectric systems [11] . Other examples for the ability to map wave phenomena among different physical systems are Zener tunnelling in optical lattices [12] , [13] , as well as the analogy between the ballistic motion of an electronic wave packet in a tight-binding lattice [14] and discrete diffraction of light in a waveguide array [15] , [16] . In this Article, we demonstrate experimentally that the ideas outlined above can be extended to the field of plasmonics [17] . For this purpose, we have fabricated arrays of evanescently coupled dielectric-loaded surface plasmon polariton waveguides (DLSPPWs) [18] , [19] by a sophisticated negative-tone gray-scale electron beam lithography process [20] . This process enables us to precisely control all geometrical sample parameters with high precision (see Methods). Thus, we can tailor the dispersion relations of the individual DLSPPWs as well as their mutual couplings in order to mimic different condensed matter phenomena. Here, we report as examples on the observation of discrete diffraction and Bloch oscillations in plasmonic systems. The complete spatial distribution of the surface plasmon polariton (SPP) intensity inside of a given waveguide array is directly monitored by leakage radiation microscopy [21] . Coupled mode theory We start by establishing the analogy between SPPs in coupled waveguide arrays (see Fig. 1a ) and electronic wave packets in crystals. Here we follow recent theoretical work [22] and describe the spatial SPP evolution in the waveguide array by the coupled mode theory (CMT) [23] . In this one-dimensional (1D) model with N waveguides, the j th waveguide ( j =1,..., N ) is characterized by its propagation constant β j and the coupling to the nearest neighbours is considered as a perturbation described by the coupling coefficients C j −1, j and C j,j +1 , respectively. The boundaries of the array are taken into account by setting C 0,1 = C N , N +1 =0. For our geometrical parameters, each DLSPPW supports a single plasmonic mode (see below). 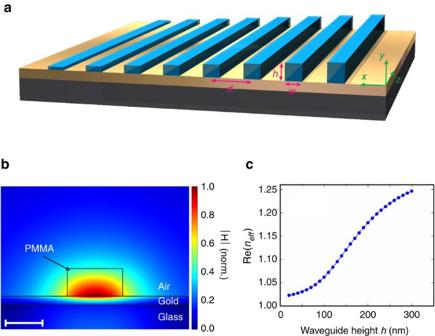Figure 1: Dielectric-loaded surface plasmon polariton waveguides. (a) Schematic view of an array of DLSPPWs on top of a thin gold film. (b) Calculated magnetic field distribution of the fundamental mode of a single DLSPPW, consisting of a PMMA ridge with widthw=300 nm and heighth=150 nm on top of a 50-nm-thin gold film. The scale bar is 200 nm. (c) Real part of the effective refractive index as a function of the DPSPPW heighth. The waveguide width is assumed to bew=300 nm in all cases. The amplitude a j ( z ) of the plasmonic mode in the j th waveguide evolves along the direction of propagation z according to: Figure 1: Dielectric-loaded surface plasmon polariton waveguides. ( a ) Schematic view of an array of DLSPPWs on top of a thin gold film. ( b ) Calculated magnetic field distribution of the fundamental mode of a single DLSPPW, consisting of a PMMA ridge with width w =300 nm and height h =150 nm on top of a 50-nm-thin gold film. The scale bar is 200 nm. ( c ) Real part of the effective refractive index as a function of the DPSPPW height h . The waveguide width is assumed to be w =300 nm in all cases. Full size image This equation of motion is completely analogous to the tight-binding model in condensed matter physics [14] . Hence, the time evolution of the crystal electron’s wavefunction can be mapped to the evolution of the SPP in coordinate space. Dielectric-loaded SPP waveguides The DLSPPWs used in our experiments consist of poly(methyl methacrylate) (PMMA) ridges that are deposited via negative-tone gray-scale electron beam lithography [20] on top of a 50-nm-thin gold film (see Methods). Figure 1b depicts the calculated magnetic field distribution of the fundamental plasmonic mode of a single DLSPPW with width w =300 nm and thickness h =150 nm at the design wavelength λ 0 =920 nm (see Methods). The magnetic field is oriented mainly along the x direction and concentrated at the PMMA–gold interface, with an evanescent decay into the gold and air. With our gray-scale lithography process, the thickness h of the PMMA ridge can be used as a parameter to conveniently adjust the DLSPPW effective refractive index in the range between n eff ≈1.05 and n eff ≈1.25 (see Fig. 1c ). Numerical calculations show that each DLSPPW supports only one single plasmonic mode at the design wavelength λ 0 =920 nm for the relevant range of waveguide heights h , if we keep the waveguide widths below w =400 nm. The coupling between adjacent DLSPPWs depends on the overlap of the evanescent field of a given DLSPPW with its neighbours. The corresponding coupling coefficients can be tailored by varying the centre-to-centre distance d between neighbouring waveguides. Discrete diffraction in plasmonic waveguide arrays In what follows, we will first discuss the case of an array of coupled DLSPPWs with nominal identical waveguide parameters and identical separations. 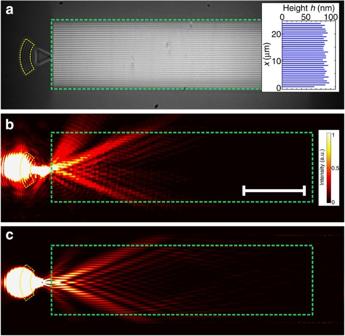Figure 2: Plasmonic discrete diffraction. (a) Micrograph of a DLSPPW array with identical waveguides. A curved grating (dashed yellow curve) and a funnel are used to excite SPPs in a single DLSPPW. The inset shows the heights of the DLSPPWs extracted from an AFM measurement. (b) Leakage radiation microscopy image showing plasmonic discrete diffraction and (c) corresponding FDTD calculation. The dashed green lines highlight the boundaries of the DLSPPW arrays. The scale bar is 20 μm. Figure 2a depicts a micrograph of such an array with a centre-to-centre distance d =750 nm. The nominal width and thickness of the individual DLSPPWs are w =300 nm and h =80 nm, respectively. The atomic force microscopy (AFM) measurement (see Methods) presented in the inset reveals only small variations of the actual waveguide thicknesses throughout the whole array. In order to excite a single DLSPPW in the middle of the array, a transverse magnetically (TM) polarized laser beam with 920-nm wavelength was focused on a curved grating coupler (see dashed yellow line). Figure 2b depicts a leakage radiation microscopy image (see Methods) of the resulting SPP intensity distribution inside the array. Starting from a single excited waveguide, the power is transferred to the neighbouring DLSPPWs by evanescent coupling of the field. These waveguides, in turn, couple to their neighbours, which results in an interference pattern with discrete maxima and minima. A major part of the intensity spreads out into two main outer lobes. This phenomenon is called discrete diffraction, as it leads to a characteristic pattern that is only found in discrete systems [3] . In the analogy to condensed matter physics, the resulting intensity pattern shows the well-known form of a quantum random walk probability distribution [24] . The edges of the array disturb the discrete diffraction pattern, as the lack of one neighbouring waveguide causes a stronger coupling of the field back into the other direction. The centre-to-centre distance d can be used to control the coupling between the DLSPPWs. By decreasing d , the power is transferred more efficiently between the waveguides. This leads to a smaller spacing between adjacent maxima and therefore a larger spreading angle of the outer lobes (see Supplementary Fig. 1 ). The discrete diffraction pattern disappears if several DLSPPWs are simultaneously excited—for example, with a Gaussian profile. For this input, the coupling of the DLSPPWs results in a beam-like spreading of the SPP intensity profile (see Supplementary Fig. 2 ). The decay length of the SPPs in the waveguides is in the order of 30 μm. This value is compatible with the assumption that the attenuation of the SPPs is dominated by absorption in the gold. In addition, leakage radiation into the glass substrate acts as another loss channel. The leakage radiation microscopy images do not indicate that the waveguide structures give rise to excessive scattering. We thus believe that scattering losses are not the limiting factor for the SPP propagation in our structures. Figure 2: Plasmonic discrete diffraction. ( a ) Micrograph of a DLSPPW array with identical waveguides. A curved grating (dashed yellow curve) and a funnel are used to excite SPPs in a single DLSPPW. The inset shows the heights of the DLSPPWs extracted from an AFM measurement. ( b ) Leakage radiation microscopy image showing plasmonic discrete diffraction and ( c ) corresponding FDTD calculation. The dashed green lines highlight the boundaries of the DLSPPW arrays. The scale bar is 20 μm. Full size image We compared our experimental results for different centre-to-centre distances and different excitation conditions both to the CMT and to full numerical calculations on the basis of the finite-difference time-domain (FDTD) method (see Methods). In all cases, we find a remarkable agreement of the calculations with the corresponding experiments. Figure 2c exemplifies the SPP intensity distribution calculated with the FDTD method, which can be directly compared with the experimental data shown in Fig. 2b . Other examples are presented in the Supplementary Fig. 3 . Bloch oscillations in plasmonic waveguide arrays By introducing a linear gradient of the effective refractive index in the transverse direction ( x direction), we can mimic the linear potential associated with a static electric field applied to a crystal. For this purpose, we fabricated DLSPPW arrays with appropriate transverse thickness profiles by varying the electron beam dose during the gray-scale lithography process. 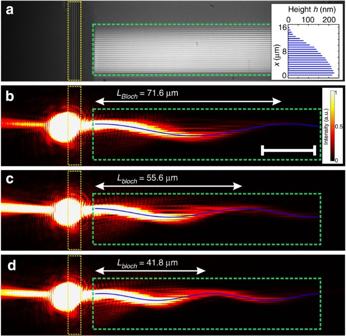Figure 3: Experimental observation of plasmonic Bloch oscillations. (a) Micrograph of a DLSPPW array with varying waveguide heights. A straight grating coupler (dashed yellow lines) is used to achieve a Gaussian input beam. The inset shows the heights of the waveguides extracted from an AFM measurement. (b–d) Leakage radiation microscopy images showing plasmonic Bloch oscillations for increasing effective index gradients. The blue curves are sinusoidal fits to the SPP intensity maxima along the propagation direction. The dashed green lines highlight the boundaries of the DLSPPW arrays. The scale bar is 20 μm. Figure 3a depicts a micrograph of such an array. We verified with AFM measurements (see inset) that the increase in the waveguide thickness Δ h and hence in the effective refractive index Δ n eff can be assumed to be linear over a reasonable part of the array. By focusing the laser on the straight grating coupler (dashed yellow line), we achieved a Gaussian intensity profile that spreads over approximately five DLSPPWs at the input of the array. The corresponding intensity distribution inside the array as monitored by leakage radiation microscopy is shown in Fig. 3b . A shape retaining oscillation of the SPP intensity distribution can clearly be observed. This oscillation is the plasmonic analogue of the Bloch oscillation of an electronic wave packet in a crystal under the influence of a static external field. The oscillation of the SPP intensity distribution is not symmetric with respect to the transverse position of the incident beam. Once the SPP wave packet is launched in the waveguide array, it is deflected downwards—that is, in the direction of the transverse refractive index gradient—reaches the maximum deflection after half a Bloch oscillation period L Bloch and is then moving back upwards to the initial transverse position. To minimize the influence of the boundaries, we have thus intentionally shifted the incident beam upwards from the middle of the array. Figure 3: Experimental observation of plasmonic Bloch oscillations. ( a ) Micrograph of a DLSPPW array with varying waveguide heights. A straight grating coupler (dashed yellow lines) is used to achieve a Gaussian input beam. The inset shows the heights of the waveguides extracted from an AFM measurement. ( b – d ) Leakage radiation microscopy images showing plasmonic Bloch oscillations for increasing effective index gradients. The blue curves are sinusoidal fits to the SPP intensity maxima along the propagation direction. The dashed green lines highlight the boundaries of the DLSPPW arrays. The scale bar is 20 μm. 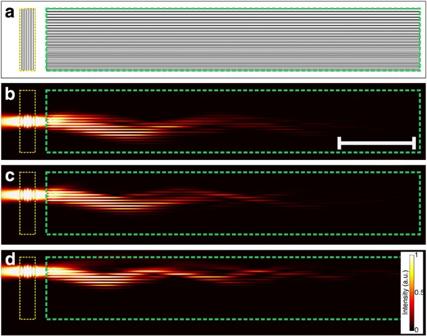Figure 4: FDTD calculations of plasmonic Bloch oscillations. (a) Sample geometry used for the simulations. (b–d) Calculated intensity distributions corresponding to the samples investigated inFig. 3b–d. The dashed green lines highlight the boundaries of the DLSPPW arrays. The scale bar is 20 μm. Full size image Figure 4 shows FDTD calculation results corresponding to the three samples investigated in Fig. 3 . The qualitative behaviour of Bloch oscillations with decreasing oscillation length is reproduced, although the calculated values are systematically smaller than the experimental ones. These differences come most likely from deviations of the actual geometrical parameters and the material properties. For example, the simulation assumes perfectly rectangular PMMA ridges, which is not given in reality. Figure 4: FDTD calculations of plasmonic Bloch oscillations. ( a ) Sample geometry used for the simulations. ( b – d ) Calculated intensity distributions corresponding to the samples investigated in Fig. 3b–d . The dashed green lines highlight the boundaries of the DLSPPW arrays. The scale bar is 20 μm. Full size image The CMT predicts that the Bloch oscillation period scales as , where is the increment of the propagation constant from one waveguide to the next [25] . Hence, L Bloch i s expected to decrease for stronger gradients of the effective refractive index. This trend can be clearly observed in the leakage radiation microscopy images presented in Fig. 3b–d , which correspond to three DLSPPW arrays with progressively larger effective refractive index gradients. For a quantitative analysis, we fitted sinusoidal functions to the intensity maxima of the leakage radiation microscopy images of the three samples. From these fits, we obtain Bloch oscillation periods of L Bloch =72 μm, L Bloch =56 μm and L Bloch =42 μm, respectively. Next, we measured the waveguide heights of all three arrays with an AFM. On the basis of these data, we calculated the effective refractive index steps from one waveguide to the next to be Δ n eff =0.011, Δ n eff =0.015 and Δ n eff =0.017, respectively. The calculated Bloch oscillation periods ( L Bloch =83 μm, L Bloch =62 μm and L Bloch =54 μm, respectively) are slightly larger than the corresponding experimental values. The corresponding Bloch oscillation periods as derived from the FDTD calculations depicted in Fig. 4 are L Bloch =50 μm, L Bloch =44 μm and L Bloch =30 μm, respectively. A summary of these values is given in Table 1 . Differences between the three values for a given array can most likely be explained by deviations of the actual waveguide profiles from a perfect rectangular shape and the slight deviations of the actual refractive index profile from a linear gradient. Moreover, an uncertainty exists in the absolute refractive index of the material from which the waveguides are made. Table 1 Bloch oscillation periods L Bloch of the three arrays. Full size table Finally, we want to estimate the number of Wannier–Stark levels that are excited by the incident Gaussian beam and hence contribute to the dynamics of the Bloch oscillation. For this purpose, we use the CMT and numerically calculate the eigenmodes of one of our DLSPPW arrays. In this step, we assume a constant increase in the effective refractive index (Δ n eff =0.0128 ⇒ L Bloch =72 μm) and a constant coupling coefficient (C=0.15 μm −1 ). Projecting the Gaussian input on the set of eigenmodes shows that approximately six Wannier–Stark levels are excited. In conclusion, we have presented the first experimental observations of discrete diffraction and Bloch oscillations of SPPs in evanescently coupled plasmonic waveguide arrays. Our experimental results are in excellent agreement with both CMT and FDTD calculations. The required gradients of the effective refractive index were realized by fabricating waveguide arrays with appropriate transverse thickness profiles via gray-scale electron beam lithography. In particular, we have demonstrated that the Bloch oscillation length can be controlled via the thickness gradient of the array. The flexibility of our fabrication approach opens new perspectives to simulate more complex solid-state phenomena, involving—for example, time-varying, random or nonlinear potentials in future experiments. Sample fabrication The samples are fabricated by evaporating 5 nm of chromium and 50 nm of gold on a glass substrate. The chromium acts as an adhesion layer and suppresses unwanted SPPs at the gold–glass interface. As a next step, a PMMA resist (MircoChem 950PMMA A4) is spin-coated on top of the gold film. At a spin speed of 1,500 r.p.m., we obtain a PMMA film thickness of ∼ 330 nm. To remove the rest of the solvent, the sample is heated for 30 min at a temperature of 175 °C. To fabricate the DLSPPW arrays, the sample is placed into an electron beam lithography system. We use a Raith Elphy nanolithography system connected to a Zeiss SIGMA scanning electron microscope for gray-scale electron beam lithography. For high electron beam doses (typical value 1,400 μC cm −2 ) and an acceleration voltage of 10 kV, the exposed PMMA resist is crosslinked and becomes resistant to solvents such as acetone. Hence, PMMA acts as a negative-tone resist in this dose range. Compared with a positive tone process, this approach has the advantage that only those areas that contain functional elements have to be exposed. The height profile of the PMMA structure can be precisely controlled via the local electron beam dose. Optical setup The optical setup consists of a 920-nm diode laser, which is TM-polarized with respect to the SPP propagation direction. The laser beam is focused with a microscope objective ( × 20 magnification, numerical aperture NA=0.4) on a SPP-grating coupler. A fraction of the excited SPP leaks through the thin gold film and couples to propagating modes in the glass substrate. This leakage radiation (as well as the directly transmitted laser beam) is collected with an oil immersion objective ( × 100 magnification, NA=1.49) and imaged on a CCD camera. Atomic force microscopy Topographical information of the DLSPPWs was obtained with AFM measurements in non-contact mode (AFM head: Solaris, probe: DCP11; both from NT-MDT). The non-contact mode was used to avoid damaging the PMMA ridge structures. Before the measurements, the AFM was re-calibrated using a calibration standard (TGZ2 from NT-MDT) with a step height of 104±2 nm. The data presented in the insets in Figs 2a and 3a are averages over 10 scanlines. Finite element method calculations We utilize the commercial software package COMSOL Multiphyics to perform a mode analysis for a single DLSPPW. The software uses the finite element method (FEM) to calculate the transverse mode profiles for a given waveguide geometry. The resulting electromagnetic field distribution and complex refractive index are analysed to study the effects of different waveguide geometries on the SPP propagation along such waveguides. FDTD calculations Full-wave numerical simulations of the actual experiment were performed by means of the FDTD method in three-dimensional (3D) space. In the FDTD method, Maxwell’s equations are discretized directly on a rectangular grid. An in-house developed code was used and calculations were performed in parallel using the message-passing interface (MPI). The geometry of the sample was extracted from AFM measurements and consists of a metal film on top of a dielectric substrate. The metal film is decorated with dielectric strips that form the DLSPPWs as well as the assisting structures that serve to couple the incident light into the DLSPPW array. A time harmonic linearly polarized Gaussian excitation was used. The metal was accounted for in the calculation by a Drude model where the free parameters are matched to guarantee an experimentally measured permittivity [26] at the operational wavelength. The intrinsic material dispersion of the waveguide material was neglected, since it is marginal and the mode dispersion is considerably stronger in each case. The spatial discretization was 10 nm. Depending on details of the samples, the spatial extent of the considered domain in our large-scale simulations was up to 113 and 34 μm in the horizontal z and x directions, respectively, and 2.3 μm in the vertical y direction. The intensity in a cross-section just above the structure was extracted at the end of the simulation from the 3D field distribution and directly compared with the experimental measurements. How to cite this article: Block, A. et al. Bloch oscillations in plasmonic waveguide arrays. Nat. Commun. 5:3843 doi: 10.1038/ncomms4843 (2014).